Reciprocal functions ofCryptococcus neoformanscopper homeostasis machinery during pulmonary infection and meningoencephalitis Copper homeostasis is important for virulence of the fungus Cryptococcus neoformans , which can cause lethal meningoencephalitis in humans. Cryptococcus cells encounter high copper levels in the lung, where infection is initiated, and low copper levels in the brain. Here we demonstrate that two Cryptococcus copper transporters, Ctr1 and Ctr4, differentially influence fungal survival during pulmonary infection and the onset of meningoencephalitis. Protein Ctr1 is rapidly degraded under the high-copper conditions found in infected lungs, and its loss has no effect in fungal virulence in mice. By contrast, deleting CTR4 results in a hypervirulent phenotype. Overexpressing either Ctr1 or Ctr4 leads to profound reductions in fungal burden in the lung. However, during the onset of meningoencephalitis, expression of the copper transporters is induced and is critical for Cryptococcus virulence. Our work demonstrates that the fungal cells switch between copper detoxification and acquisition to address different copper stresses in the host. Copper (Cu) is an essential metal for life that serves as a critical cofactor for numerous vital biological processes including oxidative stress resistance, energy production, melanin biogenesis and signal transduction [1] , [2] . The activities of proteins such as superoxide dismutase, cytochrome c oxidase, dopamine β-hydroxylase and nitrous-oxide reductase depend on Cu [1] . Moreover, numerous studies reveal the critical role of Cu for immunodefense against invading microbial pathogens. Cu-mediated pathogen killing depends on the generation of hydroxyl radicals and hydroxyl anions that causes DNA breakage, protein damage and destruction of iron–sulphur clusters [2] , [3] . Recent studies have extensively demonstrated the function of Cu as an antimicrobial agent. Levels of the mammalian Cu transporters (Ctr1 and ATP7A) in response to interferon-γ or lipopolysaccharides are markedly induced in macrophage cell lines [4] . Alveolar immune cells from mice challenged with Cryptococcus express higher Ctr1 protein levels and accumulate intracellular Cu [5] . Moreover, Cu-ionophores intensify the hostile antimicrobial Cu environment of innate immune cells in coping with C. neoformans infection [6] . As pathogens, bacterial or fungal cells lacking Cu-detoxification machinery including Cu-exporting pumps or metallothioneins (MTs) often exhibit a lower survival rate in the host [4] , [5] , [7] . Interestingly, recent work demonstrated that the disruption of Aspergillus CtpA Cu transporter causes an increased pathogenicity in the Galleria mellonella infection model [8] . C. neoformans is one of the most life-threatening human fungal pathogens and is a direct causative agent of lethal meningoencephalitis in both immunodeficient and immunocompetent individuals [9] , [10] . C. neoformans infection initiates in the human lungs, after inhalation of fungal cells from the environment. As the infection progresses, the fungal cells gradually disseminate to the brain, by uncharacterized mechanisms, where meningoencephalitis ensues [9] , [10] , [11] . Previous studies of C. neoformans virulence factors have implied that Cu plays important, but poorly characterized, roles in fungal virulence. This hypothesis is supported by the Cu dependence of many biological processes and virulence-related proteins, including melanin biogenesis, superoxide dismutase activity and Fe uptake through Cu-dependent ferroxidase activity [12] , [13] , [14] , [15] . However, recent studies also demonstrated that the Cu-detoxification proteins known as MTs are essential for fungal survival during pulmonary colonization and for virulence, indicating that C. neoformans encounters elevated Cu levels in the host early in the infectious process [5] . Here we investigate the role of two functionally redundant, high-affinity Cu + transporters (Ctr1 and Ctr4) in fungal pathogenicity in mice. We demonstrate that loss of CTR1 does not affect fungal survival in the lung because of the normally rapid degradation rate of the Ctr1 protein in a high-Cu environment similar to that found in infected lung tissues. Importantly, loss of Ctr4 results in a hypervirulent phenotype, and overexpression of CTR1 or CTR4 leads to dramatic reductions in colony forming unit (CFU), consistent with C. neoformans cells coping with high Cu levels during the initial phase of infection in the lung. Although ctr1Δctr4Δ cells also exhibit in high CFUs in the lung and brain, they do not have an impact on the survival rate of mice compared with mice infected with wild-type fungal cells. Using an intracerebral infection model to bypass lung tissue, we demonstrate that C. neoformans lacking both Ctr1 and Ctr4 exhibit strongly impaired cell growth in human cerebrospinal fluid (CSF) and reduced virulence in mouse brain. Taken together, these results demonstrate that C. neoformans senses distinct Cu environments in the lung and brain, and that the Cu acquisition machinery plays reciprocal roles in fungal virulence in these distinct niches during the course of infection. Loss of CTR4 causes hypervirulence in mice To understand the potential contribution of the Cu-acquisition machinery to C. neofomans virulence, we infected A/J mice intranasally with isogenic H99 (wild-type), ctr1Δ, ctr4Δ or ctr1Δctr4Δ strains ( Fig. 1a , Supplementary Fig. 1A and Supplementary Table ). No significant differences in survival rates were observed among the mice infected with H99, ctr1Δ or ctr1Δctr4Δ cells. However, ctr4Δ cells exhibited a strong hypervirulent phenotype. Because A/J mice carry a mutation that may be related to lung disease [16] , we further validated this result by infecting C57BL/6 mice with H99, ctr4Δ , the CTR4 complementation strain or ctr1Δctr4Δ . In agreement with the results obtained in A/J mice, ctr4Δ cells demonstrated significantly increased virulence, whereas the complementation strain showed reduced virulence compared with H99 cells ( Fig. 1b ) because of overexpressing CTR4 (discussed below). Similar survival rates were observed for mice infected with ctr1Δctr4Δ cells and mice infected with wild-type cells ( Fig. 1c ). A fungal burden analysis of the lung and brain tissues was performed in both sets of mice. We detected robust increases in the fungal burden in mice infected for ctr4Δ and ctr1Δctr4Δ , but not for mice infected with ctr1Δ cells ( Fig. 1d–g ). Because nasal mucosal membranes might capture fungal cells, resulting in uneven inoculation of fungal cells in the lung, an intratracheal infection experiment was also performed. An increased fungal burden was observed in mice infected with ctr4Δ and ctr1Δctr4Δ cells in the lung, consistent with the results for the intranasal route of infection ( Fig. 1h ). 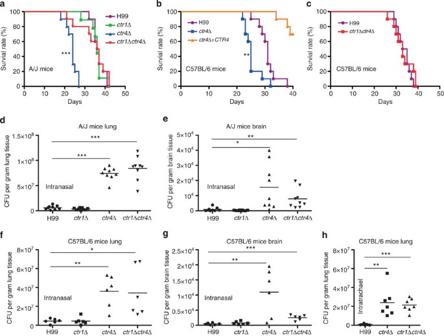Figure 1: Disruption ofCTR4increasesC. neoformansvirulence in A/J and C57BL/6 mice. (a) A/J mice (n=10) were infected intranasally with H99,ctr1Δ,ctr4Δandctr1Δctr4Δ C. neoformanscells, and the animals were monitored for signs of infection. Statistical analysis was performed using the log-rank test (***P<0.005). (b,c) C57BL/6 mice (n=10) were infected as described ina, with H99,ctr4Δ, CTR4-complemented orctr1Δctr4Δcells. Statistical analysis was performed using the log-rank test (**P<0.01). (d–h) CFUs were enumerated after 14 days of infection. CFUs were normalized to tissue weight. Statistical analysis was performed using analysis of variance (ANOVA; ***P<0.005, **P<0.01 and *P<0.05). Figure 1: Disruption of CTR4 increases C. neoformans virulence in A/J and C57BL/6 mice. ( a ) A/J mice ( n =10) were infected intranasally with H99, ctr1Δ , ctr4Δ and ctr1Δctr4Δ C. neoformans cells, and the animals were monitored for signs of infection. Statistical analysis was performed using the log-rank test (*** P <0.005). ( b , c ) C57BL/6 mice ( n =10) were infected as described in a , with H99, ctr4Δ, CTR4 -complemented or ctr1Δctr4Δ cells. Statistical analysis was performed using the log-rank test (** P <0.01). ( d – h ) CFUs were enumerated after 14 days of infection. CFUs were normalized to tissue weight. Statistical analysis was performed using analysis of variance (ANOVA; *** P <0.005, ** P <0.01 and * P <0.05). Full size image We also noted that lungs infected with ctr4Δ or ctr1Δctr4Δ were significantly enlarged, compared with those from mice infected with wild-type C. neoformans ( Fig. 2a,b ), indicating a hyperinflammatory response and greater lung tissue damage. This finding was confirmed by haematoxylin/eosin and TUNEL (terminal deoxynucleotidyl transferase dUTP nick-end labelling) staining, which showed more infiltration of mononuclear cells and higher numbers of apoptotic lung cells when mice were infected with ctr4Δ or ctr1Δctr4Δ cells as compared with the H99 strain ( Fig. 2c–f ). This lung tissue enlargement may be due to the production of a more elaborate biofilm structure by ctr4Δ and ctr1Δctr4Δ cells in the lung tissue or on blood vessels. However, no differences in biofilm formation were observed among the H99, ctr1Δ , ctr4Δ or ctr1Δctr4Δ strains ( Fig. 2g ). We also examined the CFUs in the blood, and we can only detect Cryptococcus cells in the blood, irrespective of genotype, at 21 days post infection ( Fig. 2h ), as described previously [17] . These data strongly demonstrated that the lung tissue enlargement and damage observed at 14 days post infection are due to increased fungal cell proliferation of the ctr4Δ and ctr1Δctr4Δ strains, and not enhanced biofilm formation in the lungs or blood vessels. Given that C. neoformans cells experience high Cu levels in the lung [5] , our results suggest that the loss of CTR4 efficiently reduces host killing of C. neoformans during the initial stages of infection. However, as shown in Fig. 1 , while Ctr1 and Ctr4 are independent and functionally redundant integral membrane Cu + importers, the two Cu + transporter mutants exhibit difference in pulmonary infection phenotypes in vivo . In addition, the ctr1Δctr4Δ strain exhibited increased CFUs in the lung and brain CFUs compared with the H99 strain; however, animal survival rates were indistinguishable. 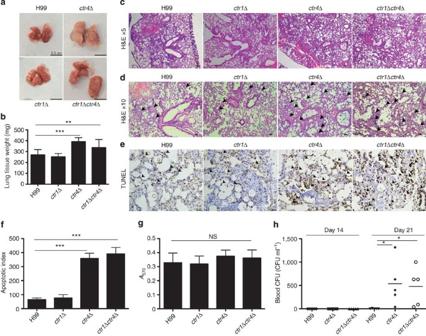Figure 2: Disruption ofCTR4induces inflammatory responses and lung damage. (a) Infected lung tissues from C57BL/6 mice were perfused, dissected and photographed after 14 days of infection (scale bar=0.5 cm). (b) Infected lung tissues (n=9) were weighed, and the data were plotted (mean, s.d.). Statistical analysis was performed using Student’st-test (***P<0.005 and **P<0.01). (c,d) Infected lung tissues from C57BL/6 mice were stained with haematoxylin and eosin and examined under a × 5 lens (c) (scale bar=100 μm) and a × 10 lens (d) (scale bar=50 μm). Arrows indicate immune cells. (e) Infected lung tissues fromcwere subjected to TUNEL staining (scale bar=25 μm). Stained cells are indicated with arrows. (f) The number of apoptotic cells of each strain was quantified. Statistical analysis was performed using Student’st-test. The data are presented as the mean±s.d. Four different microscopy views were selected and stained cells were counted (***P<0.005). (g) Biofilm formation by each strain was assayed and quantified as described previously57. Statistical analysis was performed using Student’st-test. The data are presented as the mean±s.d. (h) Enumeration of Blood CFUs. C57BL/6 mice (n=5) were infected as described inFig. 1for 14 and 21 days. Blood samples were collected and plated on SC agar plates for 3 days. Statistical analysis was performed using ANOVA (*P<0.05). Figure 2: Disruption of CTR4 induces inflammatory responses and lung damage. ( a ) Infected lung tissues from C57BL/6 mice were perfused, dissected and photographed after 14 days of infection (scale bar=0.5 cm). ( b ) Infected lung tissues ( n =9) were weighed, and the data were plotted (mean, s.d.). Statistical analysis was performed using Student’s t -test (*** P <0.005 and ** P <0.01). ( c , d ) Infected lung tissues from C57BL/6 mice were stained with haematoxylin and eosin and examined under a × 5 lens ( c ) (scale bar=100 μm) and a × 10 lens ( d ) (scale bar=50 μm). Arrows indicate immune cells. ( e ) Infected lung tissues from c were subjected to TUNEL staining (scale bar=25 μm). Stained cells are indicated with arrows. ( f ) The number of apoptotic cells of each strain was quantified. Statistical analysis was performed using Student’s t -test. The data are presented as the mean±s.d. Four different microscopy views were selected and stained cells were counted (*** P <0.005). ( g ) Biofilm formation by each strain was assayed and quantified as described previously [57] . Statistical analysis was performed using Student’s t -test. The data are presented as the mean±s.d. ( h ) Enumeration of Blood CFUs. C57BL/6 mice ( n =5) were infected as described in Fig. 1 for 14 and 21 days. Blood samples were collected and plated on SC agar plates for 3 days. Statistical analysis was performed using ANOVA (* P <0.05). Full size image Cu transporter expression dictates fungal survival in the host A deletion of the C. neoformans CTR4 gene was previously generated using an auxotrophic marker ( URA5 ) in an ura5Δ strain that was generated using 5-fluoroorotic acid (5-FOA) [18] . The ctr4Δ::URA5 (NIH) (a gift from Dr Peter Williamson, NIH, USA) and ctr4Δ::NEO strains did not exhibit capsule formation [18] or release defects ( Supplementary Fig. 1B,C ); however, the ctr4Δ::URA5 (NIH) strain did demonstrate a reduction in fungal virulence and defective cell growth under nutrient-limiting conditions [18] . To carefully verify our ctr4Δ phenotype ( ctr4Δ::NEO ), we performed Southern blot analysis of ctr4Δ::NEO and ctr1Δ::NAT ctr4Δ::NEO , which revealed a single integration of the NEO cassette at the CTR4 allele ( Supplementary Fig. 1 ). We also generated a ctr4Δ::URA5 ura5Δ::HYG strain ( Supplementary Table ) and confirmed the lack of CTR4 mRNA expression with real-time PCR ( Fig. 3b ). No differences in growth defects were observed between the wild-type strain and the isogenic Cu + transporter mutants under nutrient-deficient conditions, regardless of the addition of Cu, bathocuproine sulphonate (BCS) or uracil ( Supplementary Fig. 2A ). Although we validated the correct integration of the CTR4::URA5 cassette in our ctr4Δ::URA5 strain with integration-diagnostic PCR, we were unable to confirm correct integration in ctr4Δ::URA5 (NIH) cells ( Supplementary Fig. 3A,B ). The loss of the wild-type CTR4 allele was detected in both ctr4Δ::URA5 strains. Interestingly, we could not detect an intact ctr4Δ::URA5 allele in the CTR4 complementation strain (NIH), which should maintain URA5 at the CTR4 allele and a wild-type randomly reintegrated CTR4 allele, as mentioned previously [18] ( Supplementary Fig. 3A ). Southern blot analysis ( Supplementary Fig. 3C ) confirmed the presence of a wild-type URA5 in H99, ctr4 Δ::URA5 (NIH) and the CTR4 complementation strain (NIH), and the integration of URA5 at the CTR4 allele in the ctr4Δ::URA5 strain (NIH). However, the complementation strain does not possess a ctr4Δ::URA5 . We next determined whether the nutrient-dependent phenotype of ctr4Δ::URA5 (NIH) is because of uracil. The cell growth of ura5Δ and ctr4Δ::URA5 (NIH) was significantly inhibited when uracil was absent in the media ( Supplementary Fig. 4A ). The expression of URA5 was significantly induced in ctr4Δ::URA5 (NIH) cells in the absence of uracil, perhaps indicating that uracil starvation induces native nonfunctional URA5 in the 5′ FOA-mutagenized strain. Because we were uncertain by the genotype of the CTR4 complementation strain (NIH), we transformed a GPD promoter-CTR4HA construct into ctr4Δ::URA5 (NIH) and ctr1Δctr4Δ cells using the biolistic transformation method. CTR4HA protein expression was then examined in the resulting ctr4Δ::URA5 (NIH) GPD-CTR4HA transformant. Our data demonstrated that CTR4HA expression can complement ctr1Δctr4Δ cell growth under Cu deficiency, while ctr4Δ::URA5 (NIH) cells expressing CTR4HA retained the uracil-dependent phenotype ( Supplementary Fig. 4B ). Therefore, these analyses demonstrate that the previously used CTR4 complementation strain phenotype is not reproducible in our hands and suggest that CTR4 is not involved in general nutrient acquisition in C. neoformans ( Supplementary Figs 3 and 4 ) [18] . As our ctr4Δ::URA5 strain exhibited a trend of reduced URA5 expression and the ctr4Δ::URA5 (NIH) cells incorrectly demonstrated the CTR4 phenotype, both strains were excluded from the animal infection experiments to avoid complications in the interpretations of the results. 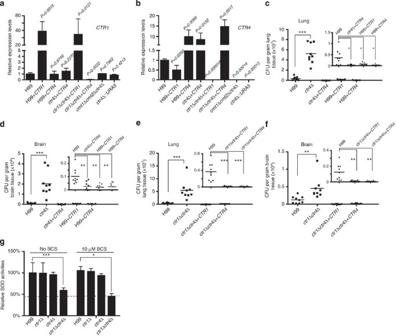Figure 3: Overexpression ofC. neoformansCu transporters impairs fungal survival in intranasal infections. (a) Strains overexpressingCTR1andCTR4were constructed. Cells were grown in SC medium for 6 h, RNA was isolated and real-time PCR was performed to quantifyCTR1expression. The data are presented as the mean±s.d. Statistical analysis was performed using Student’st-test. (b) The experiments were performed as described ina; however, primers for detectingCTR4were used. Statistical analysis was performed using Student’st-test. The data are presented as the mean±s.d. (c) Lung CFUs were enumerated from infected C57BL/6 mice as described inFig. 1d, using strains H99,ctr4Δ,ctr4Δ+CTR4, H99+CTR1and H99+CTR4.Statistical analysis was performed using ANOVA (***P<0.005, *P<0.05). CFUs of H99,ctr4Δ+CTR4, H99+CTR1and H99+CTR4are shown in the inset. (d) Brain CFUs were enumerated from infected C57BL/6 mice as described inFig. 1e, using strains H99,ctr4Δ,ctr4Δ+CTR4, H99+CTR1and H99+CTR4. Statistical analysis was performed using ANOVA (***P<0.005, **P<0.01). CFUs for H99,ctr4Δ+CTR4, H99+CTR1and H99+CTR4are shown in the inset. (e) Lung CFUs were enumerated from infected C57BL/6 mice as described inFig. 1dusing strains H99,ctr1Δctr4Δ,ctr1Δctr4Δ+CTR1andctr1Δctr4Δ+CTR4. Statistical analysis was performed using ANOVA (***P<0.005). CFUs for H99,ctr1Δctr4Δ+CTR1andctr1Δctr4Δ+CTR4are shown in the inset. (f) Brain CFUs were enumerated from infected C57BL/6 mice as described inFig. 1dusing strains H99,ctr1Δctr4Δ,ctr1Δctr4Δ+CTR1andctr1Δctr4Δ+CTR4. Statistical analysis was performed using ANOVA (**P<0.01). CFUs for H99,ctr1Δctr4Δ+CTR1andctr1Δctr4Δ+CTR4are shown in the inset. (g) Cells were grown in SC medium or SC medium supplemented with 10 μM BCS for 6 h. Total protein was isolated and SOD activity was measured. Statistical analysis was performed using Student’st-test. The data are presented as the mean±s.d. Figure 3: Overexpression of C. neoformans Cu transporters impairs fungal survival in intranasal infections. ( a ) Strains overexpressing CTR1 and CTR4 were constructed. Cells were grown in SC medium for 6 h, RNA was isolated and real-time PCR was performed to quantify CTR1 expression. The data are presented as the mean±s.d. Statistical analysis was performed using Student’s t -test. ( b ) The experiments were performed as described in a ; however, primers for detecting CTR4 were used. Statistical analysis was performed using Student’s t -test. The data are presented as the mean±s.d. ( c ) Lung CFUs were enumerated from infected C57BL/6 mice as described in Fig. 1d , using strains H99, ctr4Δ , ctr4Δ + CTR4 , H99+ CTR1 and H99 +CTR4. Statistical analysis was performed using ANOVA (*** P <0.005, * P <0.05). CFUs of H99, ctr4Δ + CTR4 , H99+ CTR1 and H99 +CTR4 are shown in the inset. ( d ) Brain CFUs were enumerated from infected C57BL/6 mice as described in Fig. 1e , using strains H99, ctr4Δ , ctr4Δ+CTR4 , H99+ CTR1 and H99 +CTR4 . Statistical analysis was performed using ANOVA (*** P <0.005, ** P <0.01). CFUs for H99, ctr4Δ+CTR4 , H99+ CTR1 and H99 +CTR4 are shown in the inset. ( e ) Lung CFUs were enumerated from infected C57BL/6 mice as described in Fig. 1d using strains H99, ctr1Δctr4Δ , ctr1Δctr4Δ + CTR1 and ctr1Δctr4Δ + CTR4 . Statistical analysis was performed using ANOVA (*** P <0.005). CFUs for H99, ctr1Δctr4Δ + CTR1 and ctr1Δctr4Δ + CTR4 are shown in the inset. ( f ) Brain CFUs were enumerated from infected C57BL/6 mice as described in Fig. 1d using strains H99, ctr1Δctr4Δ , ctr1Δctr4Δ + CTR1 and ctr1Δctr4Δ + CTR4 . Statistical analysis was performed using ANOVA (** P <0.01). CFUs for H99, ctr1Δctr4Δ + CTR1 and ctr1Δctr4Δ + CTR4 are shown in the inset. ( g ) Cells were grown in SC medium or SC medium supplemented with 10 μM BCS for 6 h. Total protein was isolated and SOD activity was measured. Statistical analysis was performed using Student’s t -test. The data are presented as the mean±s.d. Full size image As shown in Fig. 1 , the CTR4 complementation strain was less virulent than the isogenic H99 strain. Quantitative reverse transcription–PCR (qRT–PCR) analysis revealed that expression of CTR4 in the complemented strain was higher than that in the wild-type; therefore, we hypothesised that the reduced virulence phenotype was because of the overexpression of CTR4 . To test this hypothesis, we overexpressed CTR1 or CTR4 in the H99 or ctr1Δctr4Δ strains, respectively. All strains overexpressing the Cu transporters were used for fungal burden analysis ( Fig. 3a,b ). We showed that all strains with higher expression of either the Ctr1 or Ctr4 Cu transporter had significantly reduced fungal burdens in lung and brain tissues ( Fig. 3c–f ). Previous inductively coupled plasma mass spectrometry analysis suggested that the ctr4Δ::URA5 (NIH) strain exhibited higher cell-associated Cu levels than wild-type cells, implying that the ctr4Δ::URA5 (NIH) strain has more bioavailable intracellular Cu [18] . However, the inductively coupled plasma mass spectrometry (ICP-MS) method quantifies Cu from whole cells and does not necessarily reflect intracellular Cu status. Moreover, the pleiotropic growth phenotype observed for the ctr4Δ::URA5 (NIH) strain is independent of CTR4 ( Supplementary Figs 3 and 4 ) [18] . To determine the contribution of the C. neoformans Cu + transporters to intracellular Cu availability, we assayed the activity of Cu/Zn-superoxide dismutase (SOD) in wild-type and Cu + transporter mutant strains because Cu/Zn-SOD activity depends on the amount of bioavailable intracellular Cu [19] . Although the Cu/Zn-SOD activities of the H99, ctr1Δ and ctr4Δ strains were similar, that of the ctr1Δctr4Δ strain was significantly reduced by 40% in SC medium and >50% in the medium that was Cu-limited by addition of the extracellular Cu + chelator, BCS ( Fig. 3g ), indicating that CTR1 and CTR4 are functionally independent Cu + importers and that the disruption of either Cu transporter does not significantly influence intracellular Cu status. CTR4 has been shown to negatively regulate the expression of C. neoformans MTs; however, it is not clear whether the pyrimidine biosynthesis pathway, or the Ctr4 Cu + transporter, influences expression of MTs [18] . In our hands, expression of both CMT1 and CMT2 are significantly reduced in the absence of CTR4 when cells encountered high-Cu conditions and in the lungs ( Fig. 4a,b ), consistent with CTR4 encoding a high-affinity Cu + importer in C. neoformans . To determine whether the hypervirulent phenotype of ctr4Δ is due to the modulation of expression of CMTs , as shown previously [18] , we deleted CTR4 in the cmt1Δcmt2Δ strain ( Supplementary Table and Fig. 4c,d ). The cmt1Δcmt2Δctr4Δ strain did not exhibit a nutrient-dependent phenotype ( Supplementary Fig. 2B ). Intranasal infection and the fungal burden analysis revealed that fungal colonization was reduced in the lungs and brains of mice infected with cmt1Δcmt2Δ ( Fig. 4c,d ). Deleting CTR4 in the cmt1Δcmt2Δ strain rescued the survival of cmt1Δcmt2Δ cells in the lung and brain to near wild-type levels ( Fig. 4c,d ), demonstrating that Ctr4 independently regulates fungal virulence, regardless of the presence of MTs. 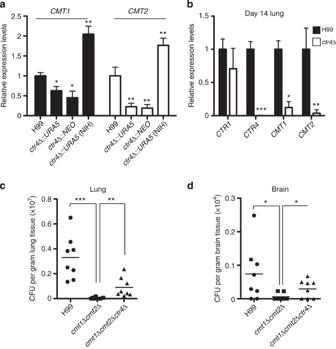Figure 4: Ctr4 modulates fungal virulence independently of the regulation of metallothioneins. (a)C. neoformansH99,ctr4Δ::URA5, ctr4Δ::NEO, ctr4Δ::URA5(NIH) cells were subcultured in SC medium supplemented with 30 μM Cu for 3 h. RNA was isolated and real-time PCR was performed to detectCMT1,CMT2andACT1.Statistical analysis was performed using Student’st-test. The data are presented as the mean±s.d. (b) C57BL/6 mice were intranasally infected with H99 orctr4Δ::NEOcells for 7 days. RNA was isolated as described previously30. Real-time PCR was performed to detectCTR1, CTR4, CMT1,CMT2andACT1.Statistical analysis was performed using Student’st-test. The data are presented as the mean±s.d. (c,d) CFU analysis were performed as described inFig. 1d. Statistical analysis was performed using ANOVA (***P<0.005, **P<0.01 and *P<0.05). Figure 4: Ctr4 modulates fungal virulence independently of the regulation of metallothioneins. ( a ) C. neoformans H99, ctr4Δ::URA5, ctr4Δ::NEO, ctr4Δ::URA5 (NIH) cells were subcultured in SC medium supplemented with 30 μM Cu for 3 h. RNA was isolated and real-time PCR was performed to detect CMT1 , CMT2 and ACT1. Statistical analysis was performed using Student’s t -test. The data are presented as the mean±s.d. ( b ) C57BL/6 mice were intranasally infected with H99 or ctr4Δ::NEO cells for 7 days. RNA was isolated as described previously [30] . Real-time PCR was performed to detect CTR1, CTR4, CMT1 , CMT2 and ACT1. Statistical analysis was performed using Student’s t -test. The data are presented as the mean±s.d. ( c , d ) CFU analysis were performed as described in Fig. 1d . Statistical analysis was performed using ANOVA (*** P <0.005, ** P <0.01 and * P <0.05). Full size image The Ctr1 and Ctr4 proteins have distinct properties Our data demonstrated that the ctr1Δ strain does not exhibit changes in fungal virulence but that strains overexpressing CTR1 results in decreased fungal burden. One possible explanation is that Ctr1 is rapidly degraded in the presence of high Cu levels. We measured the Ctr1 protein half-life under Cu-depleted conditions. To eliminate the effect of the overexpression system on the protein-level quantification, we generated integration cassettes that insert a DNA sequence encoding a HA tag before the stop codon in the genes of interests to compare the proteins expressed from their native loci ( Fig. 5a ). We first repressed or induced protein expression by culturing cells in the presence of Cu or BCS, respectively, and robust protein expression was detected for both the Ctr1 and Ctr4 proteins under low-Cu conditions and for Cmt1 under high-Cu conditions ( Fig. 5b and Supplementary Fig. 5A ). We then extensively induced the expression of CTR1HA and CTR4HA in the presence of 1 mM BCS for 6 h and measured the Ctr1HA and Ctr4HA protein stability in response to high Cu levels. As shown in Fig. 5c and Supplementary Fig. 5B , the Ctr1HA protein was not detected after a 5-min exposure to Cu, whereas Ctr4HA was maintained for at least 90 min after Cu addition. These data strongly suggest that, in contrast to Ctr4, the Ctr1 protein is highly unstable under high-Cu conditions. To ascertain whether Ctr1 is expressed in the lung, we performed immunohistochemistry. Although expression of Cmt1HA and Ctr4HA was detected 2 days post infection, we detected little to no signal for Ctr1HA ( Fig. 5d ). 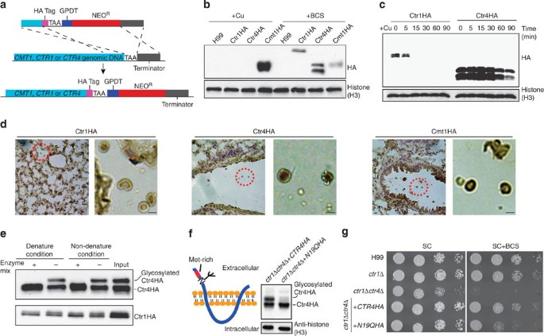Figure 5:C. neoformansCu transporters have distinct properties. (a) A DNA sequence encoding the HA tag was integrated before the stop codon ofCTR1andCTR4. Sequences upstream and downstream ofCTR1,CTR4orCMT1were cloned into a plasmid containing HA tag construct. The resulting plasmid was amplified and integrated into the genome of the H99 strain to generate strainsCTR1HA,CTR4HAorCMT1HA. (b) Cells were grown in SC medium supplemented with 200 μM BCS or 200 μM Cu for 6 h. Proteins were isolated and probed with the anti-HA and anti-histone H3 antibodies (seeSupplementary Fig. 5Afor full blots). (c) Cells were grown in SC medium supplemented with 1 mM BCS for 6 h and washed three times with H2O. The cells were then treated with 100 μM Cu. Proteins were isolated at different time points and probed with the anti-HA and anti-histone H3 antibodies (seeSupplementary Fig. 5Bfor full blots). (d) C57BL/6 mice were infected withC. neoformanscells expressingCTR1HA,CTR4HAandCMT1HA. Two days post infection, lung tissues were removed and subjected to immunohistochemical anlaysis (scale bar=50 μm). Red circles indicateC. neoformanscells, which are shown in the right panels (scale bar=25 μm). (e) The expression of the Ctr1 and Ctr4 Cu+transporters was induced by culturing cells in SC medium supplemented with 1 mM BCS for 6 h. Proteins were then isolated and mixed with protein deglycosylation mix (NEB) for 4 h. Proteins were separated on a 15% SDS–PAGE gel and an anti-HA antibody was used to detect Ctr4HA and Ctr1HA (seeSupplementary Fig. 5Cfor full blots). (f) The transmembrane domains of Ctr4 were predicted using TMHMM 2.0 (http://www.cbs.dtu.dk/services/TMHMM-2.0) (left panel). Ctr4 Asn19 was mutated to Gln using a PCR-based approach and the mutatedCTR4genomic DNA sequence was integrated into theCTR4-native allele. The protein was isolated and probed with an anti-HA antibody (seeSupplementary Fig. 5Dfor full blots). (g)ctr1Δctr4Δcells expressing wild-typeCTR4HAand the N19QHA mutation were spotted on SC agar supplemented with 125 μM BCS. Images were acquired after a 2-day incubation at 30 °C. Figure 5: C. neoformans Cu transporters have distinct properties. ( a ) A DNA sequence encoding the HA tag was integrated before the stop codon of CTR1 and CTR4 . Sequences upstream and downstream of CTR1 , CTR4 or CMT1 were cloned into a plasmid containing HA tag construct. The resulting plasmid was amplified and integrated into the genome of the H99 strain to generate strains CTR1HA , CTR4HA or CMT1HA . ( b ) Cells were grown in SC medium supplemented with 200 μM BCS or 200 μM Cu for 6 h. Proteins were isolated and probed with the anti-HA and anti-histone H3 antibodies (see Supplementary Fig. 5A for full blots). ( c ) Cells were grown in SC medium supplemented with 1 mM BCS for 6 h and washed three times with H 2 O. The cells were then treated with 100 μM Cu. Proteins were isolated at different time points and probed with the anti-HA and anti-histone H3 antibodies (see Supplementary Fig. 5B for full blots). ( d ) C57BL/6 mice were infected with C. neoformans cells expressing CTR1HA , CTR4HA and CMT1HA . Two days post infection, lung tissues were removed and subjected to immunohistochemical anlaysis (scale bar=50 μm). Red circles indicate C. neoformans cells, which are shown in the right panels (scale bar=25 μm). ( e ) The expression of the Ctr1 and Ctr4 Cu + transporters was induced by culturing cells in SC medium supplemented with 1 mM BCS for 6 h. Proteins were then isolated and mixed with protein deglycosylation mix (NEB) for 4 h. Proteins were separated on a 15% SDS–PAGE gel and an anti-HA antibody was used to detect Ctr4HA and Ctr1HA (see Supplementary Fig. 5C for full blots). ( f ) The transmembrane domains of Ctr4 were predicted using TMHMM 2.0 ( http://www.cbs.dtu.dk/services/TMHMM-2.0 ) (left panel). Ctr4 Asn19 was mutated to Gln using a PCR-based approach and the mutated CTR4 genomic DNA sequence was integrated into the CTR4 -native allele. The protein was isolated and probed with an anti-HA antibody (see Supplementary Fig. 5D for full blots). ( g ) ctr1Δctr4Δ cells expressing wild-type CTR4HA and the N19QHA mutation were spotted on SC agar supplemented with 125 μM BCS. Images were acquired after a 2-day incubation at 30 °C. Full size image Interestingly, we detected two protein species for both Cu transporters ( Fig. 5b, c , Supplementary Fig. 5A,B ), suggesting that these Cu + transporters undergo post-translational modification. In mammals, the Ctr1 Cu + transporter is glycosylated at two positions within the N terminus [20] , [21] , [22] , [23] . We used a protein deglycosylation enzyme mix that removes both N- and O-glycosylation to determine whether C. neoformans Cu transporters are glycosylated. After incubation, we were unable to detect the upper band for Ctr4HA, suggesting that Ctr4 is glycosylated. Experimental results under identical conditions gave no evidence that Ctr1 is glycosylated ( Fig. 5e and Supplementary Fig. 5C ). The prediction algorithms from the NetNGlyc and NetOGlyc web servers showed that the Asn19 residue on Ctr4 is a potential N-glycosylation site. A candidate glycosylation-resistant mutant was generated by integrating a mutated DNA sequence at the CTR4 -native allele ( Supplementary Fig. 6A ). Correct integration was confirmed with PCR ( Supplementary Fig. 6A ) and gene copy tests with real-time PCR ( Supplementary Fig. 6B ). The immunoblot analysis demonstrated that mutating Asn19 completely abolishesd the glycosylation of Ctr4HA ( Fig. 5f and Supplementary Fig. 5D ). Furthermore, the glycosylation mutant rescued the ctr1Δctr4Δ growth phenotype in the presence of BCS, although not to the level of the wild-type CTR4 complementation strain ( Fig. 5g ), suggesting that fully functional Ctr4 requires glycosylation. As protein glycosylation is processed on endoplasmic reticulum (ER) and may affect protein trafficking, we performed indirect immunofluorescence assays and observed plasma membrane and ER-associated protein localization for both the wild-type Ctr4 and N19Q-mutant proteins, suggesting that Ctr4 trafficking is not dependent on N19 glycosylation ( Supplementary Fig. 6C ). Ctr1 and Ctr4 are critical during meningoencephalitis Although the ctr1Δctr4Δ -mutant strain exhibited higher fungal burden in the lung and brain, surprisingly, identical survival was observed in mice infected with ctr1Δctr4Δ or H99 cells ( Fig. 1a ). We hypothesized that ctr1Δctr4Δ cells counter Cu toxicity in the lung, leading to high fungal intrusion into the brain, where Cu transporters are required for virulence. To test this hypothesis, we employed ex vivo two-photon microscopy analysis of lung and brain tissues to examine the fluorescence intensity of green fluorescent protein (GFP) that is driven by either the CTR4 or CMT1 promoters. One and seven days post intranasal or intracerebral infection, the CMT1p-GFP produced higher GFP signals in the lung than that of CTR1p-GFP and CTR4p-GFP ( Fig. 6a ), as previously described [5] . In the brain, the fluorescence intensities of CTR1p-GFP and CTR4p-GFP were higher than that of CMT1p-GFP ( Fig. 6b ). These data strongly suggest that C. neoformans cells sense Cu-limitation conditions in the host brain. In human CSF, the copper level is ~7.5±3.1 ng ml −1 (~0.12±0.048 nmol ml −1 ) [24] . As access to the host CSF is critical for cryptococcosis , we examined fungal cell growth in human CSF with or without the supplementation of Cu. CFU analysis indicated that the growth of the C. neoformans Cu-acquisition mutant ( ctr1Δctr4Δ ) was strongly limited in the absence of exogenous Cu ( Fig. 6c ). Interestingly, the addition of Cu also stimulated the growth of wild-type cells after 96-h incubation, indicating that Cu is important for C. neoformans to survival in the CSF. 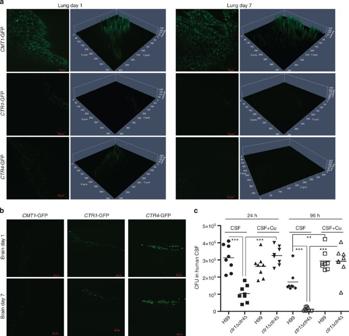Figure 6:C. neoformanssenses Cu deficiency in the host brain and human CSF. (a) C57BL/6 mice were intranasally infected withC. neoformanscells expressingCMT1p-GFP,CTR1p-GFPorCTR4p-GFP. After days 1 and 7, lung tissues were removed and analysed by two-photon microscopy with a × 10 lens (scale=50 μm), and the 2.5-D analysis was performed using the ZEN2012 software to quantify GFP signal intensities in the lung. (b) C57BL/6 mice were intracerebrally infected withC. neoformanscells expressingCMT1p-GFP,CTR1p-GFPorCTR4p-GFP.After days 1 and 7, the brain was removed and examined using a × 10 lens with a 4.0 magnification factor (scale=20 μm). (c) Human CSF was inoculated withC. neoformanscells H99 andctr1Δctr4. CFUs were enumerated as described previously56. Figure 6: C. neoformans senses Cu deficiency in the host brain and human CSF. ( a ) C57BL/6 mice were intranasally infected with C. neoformans cells expressing CMT1p-GFP , CTR1p-GFP or CTR4p-GFP . After days 1 and 7, lung tissues were removed and analysed by two-photon microscopy with a × 10 lens (scale=50 μm), and the 2.5-D analysis was performed using the ZEN2012 software to quantify GFP signal intensities in the lung. ( b ) C57BL/6 mice were intracerebrally infected with C. neoformans cells expressing CMT1p-GFP , CTR1p-GFP or CTR4p-GFP. After days 1 and 7, the brain was removed and examined using a × 10 lens with a 4.0 magnification factor (scale=20 μm). ( c ) Human CSF was inoculated with C. neoformans cells H99 and ctr1Δctr4 . CFUs were enumerated as described previously [56] . Full size image To bypass the lung, mice were infected intracerebrally with H99, ctr1Δ , ctr4Δ and ctr1Δctr4Δ strains. Mice infected with H99, ctr1Δ and ctr4Δ exhibited similar survival rates, while the ctr1Δctr4Δ strain exhibited a significant reduction in fungal virulence ( Fig. 7a ), indicating that either of the functionally redundant Ctr1 or Ctr4 Cu + importers is required for C. neoformans survival in the brain. To further address the Cu environment that is sensed by C. neoformans in brain tissue, we injected mice with H99, cmt1Δcmt2Δ or ctr1Δctr4Δ and demonstrated that MTs play no role in C. neoformans survival in the brain ( Fig. 7b ). These data suggest that C. neoformans cells do not experience a Cu toxicity environment, but rather a Cu-deficient environment in the brain that limits virulence. When a higher fungal cell inoculum was used for intracerebral infection of ctr1Δctr4Δ , increased fungal virulence was observed (compare Fig. 7b,c ), which may explain the difference in the survival rates of mice infected with H99 and ctr1Δctr4Δ in Fig. 1a . Given that intranasal infection with ctr1Δctr4Δ produced a fivefold increase in CFUs in the brain compared with infection with H99 ( Fig. 1 ), these observations support the hypothesis that the low-Cu conditions of the brain inhibit fungal cell proliferation of ctr1Δctr4Δ , resulting in similar animal death rates. It has been shown that in response to interferon (IFN)-γ activation, macrophages robustly express the mammalian Ctr1 Cu + transporter and accumulate antimicrobial Cu in the phagosomal compartment [4] , [25] . To further analyse immune responses in the lung and brain, we measured the production of two important cytokines (IFN-γ and tumour necrosis factor (TNF-α) after 7 or 14 days in uninfected mice and mice intranasally infected with C. neoformans . We show here that IFN-γ and TNF-α were significantly increased in response to C. neoformans infection in the lung, whereas their levels remained constant in the brain ( Fig. 7d ). 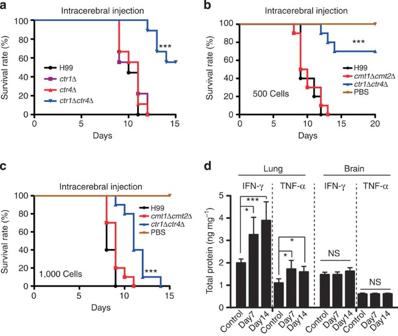Figure 7:C. neoformansCu+transporters are required for meningoencephalitis. (a) C57BL/6 mice (n=9) were infected intracerebrally with H99,ctr1Δ,ctr4Δandctr1Δctr4Δcells, and the animals were monitored for signs ofC. neoformansinfection. Statistical analysis was performed using the log-rank test (***P<0.005). (b,c) Experiments were performed as described ina. EachC. neoformansstrain was used to infect 10 C57BL/6 mice. Statistical analysis was performed using the log-rank test (***P<0.005). (d) C57BL/6 mice (n=4) were infected intranasally with H99 for 7 and 14 days. The control mice (n=4) were not infected. Lung and brain tissues were harvested, and proteins were isolated and quantified. IFN-γ and TNF-α ELISA assays were performed. Statistical analysis was performed using Student’st-test. The data are presented as the mean±s.d. Figure 7: C. neoformans Cu + transporters are required for meningoencephalitis. ( a ) C57BL/6 mice ( n =9) were infected intracerebrally with H99, ctr1Δ , ctr4Δ and ctr1Δctr4Δ cells, and the animals were monitored for signs of C. neoformans infection. Statistical analysis was performed using the log-rank test (*** P <0.005). ( b , c ) Experiments were performed as described in a . Each C. neoformans strain was used to infect 10 C57BL/6 mice. Statistical analysis was performed using the log-rank test (*** P <0.005). ( d ) C57BL/6 mice ( n =4) were infected intranasally with H99 for 7 and 14 days. The control mice ( n =4) were not infected. Lung and brain tissues were harvested, and proteins were isolated and quantified. IFN-γ and TNF-α ELISA assays were performed. Statistical analysis was performed using Student’s t -test. The data are presented as the mean±s.d. Full size image Human pathogenic fungi adapt to distinct environments by rapidly altering gene expression in response to environmental stimuli. To survive, replicate and invade host tissues, pathogenic fungi have evolved efficient and sophisticated machineries to compete for essential nutrients, including metals. In the last decade, studies have implied that Cu is a key virulence modulator for C. neoformans and is required for fungal virulence [13] , [14] , [18] , [26] , [27] , [28] . Fungal pathogens require Cu for maintaining normal cell growth and are equipped with Cu-detoxification defences, suggesting the possibility that fungal cells encounter both Cu scarcity and toxicity during their infectious life cycles. The regulation of Cu acquisition and detoxification is mediated by the transcription factor, Cuf1. The first report of the regulation of Cu homeostasis by Cuf1, published by in ref. 29 , revealed that a cuf1Δ strain is sensitive to both low and high Cu [12] , [29] . A subsequent study showed that Cuf1 controls the expression of the Cu transporter CTR4 and that the cuf1Δ strain is avirulent in a tail vein infection model, thus suggesting that Cu acquisition is essential for C. neoformans virulence in mice [18] , [27] . However, recent work has demonstrated that Cuf1 activates both the Cu-detoxification machinery and the Cu-acquisition machinery, in response to high or low Cu conditions, respectively [12] . Moreover, although C. neoformans senses high Cu in the lung and Cu-detoxification genes are critical for fungal survival in the lung, CTR4 is still expressed in the lung at relatively low levels [5] , [18] , [30] . What roles does C. neoformans Cu homeostasis play during fungal infection? C. neoformans possesses two high-affinity Cu + importers (Ctr1 and Ctr4) belonging to the Ctr family, which is conserved from yeast to mammals [12] . The Ctr family forms homotrimer structures to generate a Cu + -importing channel [1] , [31] . Ctr1 and Ctr4 are independent and functionally redundant Cu + importers whose expression is regulated by Cu [12] , [32] . The recently published nutrient-dependent phenotype of the C. neoformans ctr4Δ mutant is of great interest but unexpected [18] , and this phenotype has never been observed in other organisms, including Saccharomyces cerevisiae , Candida albicans , Schizosaccharomyces pombe , Aspergillus fumigatus, Drosophila and mice [8] , [33] , [34] , [35] , [36] , [37] . Interestingly, the nutrient phenotype of CTR4 in C. neoformans has not been reported in other studies. For example, two independent studies demonstrated robust cell growth of cuf1Δ strains under nutrient-deficient condition [12] , [32] , given Cuf1 is a positive regulator of CTR4 (ref. 12 , 27 ). The nutrient phenotype of the ctr4Δ strain has not been reproduced while generating the ctr4Δ mutant using other markers, such as NEO , HYG or URA5 ( Supplementary Table , Figs 1 and 4 , Supplementary Figs 2 and 3 ) [12] . Generating mutants using the URA cassette and a parent strain obtained from 5-FOA mutagenesis are not optimal because previous reports have demonstrated that the ura mutant affects fungal virulence, colony morphology and biofilm formation [38] , [39] , [40] , [41] , [42] . The reintegration of wild-type URA at other chromosomal loci does not fully reverse the phenotype and activity of orotidine 5-phosphate decarboxylase [39] , [40] , [41] , [42] . In our hands, the ctr4Δ::URA5 (NIH) strain exhibited a uracil-dependent phenotype. Moreover, expressing GPD-CTR4HA in this strain did not complement the phenotype ( Supplementary Fig. 4 ). Because C. neoformans senses elevated Cu levels in the lung, Ctr4 negatively regulates C. neoformans virulence during pulmonary infection, leading to a remarkable induction of fungal growth, hyperinflammatory responses and severe lung cell damage ( Figs 1 and 2 ). The greater fitness of ctr4Δ and ctr1Δctr4Δ cells in lung tissue results in the increased dissemination of fungal cells into brain tissue. Furthermore, overexpressing the Ctr1 or Ctr4 Cu transporters greatly enhances fungal killing by pulmonary antimicrobial Cu, strongly indicating that Cu transporters negatively influence fungal virulence in the lung ( Fig. 3 ). A Ctr4 mutant has been shown to accumulate Cu and affect MT expression [18] , although it is unclear whether the induction of MTs is because of pyrimidine biosynthesis or Ctr4. In S. cerevisiae , the disruption of Cu importers reduces the activation of the MT promoter under high-Cu conditions [43] . In the present study, deleting C. neoformans CTR4 reduces the expression of MTs both in vitro and vivo , demonstrating that deleting the high-affinity Cu + importer CTR4 reduces the activation of Cu-detoxification machinery ( Fig. 4a,b ). Irrespective of how CTR4 modulates the expression of MTs, the hypervirulent phenotype of ctr4Δ is not because of the induction of MTs ( Fig. 4c,d ). In the present work, differing levels of protein stability and post-translational modification of Ctr1 and Ctr4 were observed. While ctr1Δ does not affect animal survival or CFUs relative to the wild-type parental strain ( Fig. 1 ), Ctr1 is extremely unstable in the presence of exogenous Cu and in the lung ( Fig. 5c,d ). Interestingly, a strong candidate for an N-glycosylation site was detected in Ctr4 near the putative amino-terminal extracellular domain Cu-binding motifs. The glycosylation of Ctr4 resembles that of mammalian Ctr1, in which glycosylation influences Cu uptake [20] . Although the N19Q mutant restored Cu uptake in ctr1Δctr4Δ cells, complemented cells exhibited reduced growth compared with ctr1Δctr4Δ cells expressing wild-type CTR4 , implying that N-glycosylation is involved in facilitating Ctr4 function in an undefined manner. Ctr4 has been hypothesized to be important for cryptococcal meningoencephalitis [18] , [27] . Our results provide the first evidence that C. neoformans switches from Cu detoxification to acquisition modes when it disseminates from the lung to the brain ( Fig. 8a ). The increased fitness of ctr4Δ and ctr1Δctr4Δ cells in the lung leads to a higher fungal proliferation, which, in turns, increases infiltration of fungal cells into the brain, where C. neoformans requires Cu ( Fig. 8b ). Because the ctr4Δ strain contains a functional Ctr1 Cu + transporter, ctr4Δ cells are able to efficiently acquire Cu from the brain, leading to a hypervirulent phenotype ( Fig. 8b ). Although the number of ctr1Δctr4Δ cells in the brain is increased compared with the wild-type H99, the Cu-deficient environment in the brain does not permit the robust growth of ctr1Δctr4Δ cells ( Fig. 8b ). Interestingly, infection routes determine the virulence phenotype of ctr1Δctr4Δ , implying that entry rather than replication of C. neoformans in the brain is critical for fungal virulence in the mouse model [44] , [45] . Because the ctr1Δctr4Δ strain remains virulent in the intracerebral infection model, we speculate that there are other Cu uptake machineries in C. neoformans that are active in Cu transport during the formation of meningoencephalitis. 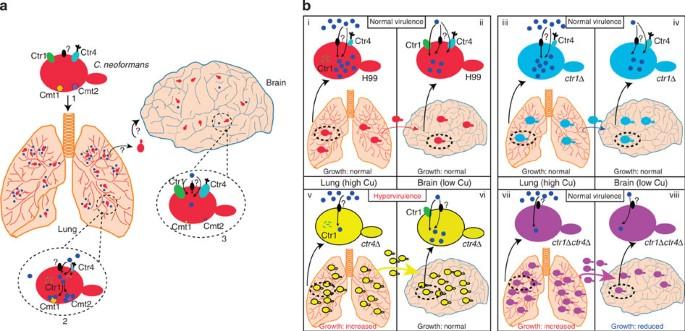Figure 8: A model of the function of theC. neoformansCu homeostasis machinery during systemic infection. (a) Model of the roles of Cu transporters duringC. neoformansinfection. (1) AC. neoformanscell possesses Cu-acquisition (Ctr1 and Ctr4) and Cu-detoxification (Cmt1 and Cmt2) proteins. (2) During pulmonary infection,C. neoformanssenses a high-Cu environment. Ctr1 is quickly degraded, but Ctr4 is still expressed. Cmt1 and Cmt2 are expressed to protect fungal cells from antimicrobial Cu in the host lung. (3) During meningoencephalitis,C. neoformansutilizes Ctr1 and Ctr4 for Cu uptake, whereas the expression of Cmt1 and Cmt2 is reduced and therefore these proteins play no function in the brain. We speculate that there are uncharacterized Cu transport machineries inC. neoformans, such as low-affinity or nonspecific transporters. (b) Models of the phenotypes ofC. neoformanstransporter mutantsin vivo. (i) The wild-type strain degrades the Ctr1 Cu+transporter in the lung, while Ctr4 is active and transports the host antimicrobial Cu. (ii) In the brain, Ctr1 and Ctr4 are expressed for Cu acquisition. (iii and iv) In thectr1Δstrain, the functionally redundant Cu+ transporter Ctr4 can transport Cu in both the lung and brain, enabling growth in both tissues similar to that observed for wild-typeC. neoformans.(v) Thectr4Δstrain exhibits increased fungal proliferation in the lung due to the fast protein degradation of Ctr1 and the disruption ofCTR4, leading to increased dissemination of fungal cells into the brain. (vi) Because the functionally redundant Cu+transporter Ctr1 is expressed inctr4Δcells and the number ofctr4Δcells in the brain is increased, thectr4Δstrain exhibits increased fungal virulence. (vii) The cell growth of thectr1Δctr4Δstrain is increased in the lung, resembling that of thectr4Δstrain, resulting in increased dissemination of fungal cells in the brain. (viii) Owing to the lack of functional Cu+transporters in thectr1Δctr4Δstrain, the cell growth is inhibited in the brain. Therefore, the Cu-replete environment in the lung and Cu-deficient conditions in the brain generates a Cu-balance for thectr1Δctr4Δstrain, resulting in a survival rate equal to that of the wild type. Figure 8: A model of the function of the C. neoformans Cu homeostasis machinery during systemic infection. ( a ) Model of the roles of Cu transporters during C. neoformans infection. (1) A C. neoformans cell possesses Cu-acquisition (Ctr1 and Ctr4) and Cu-detoxification (Cmt1 and Cmt2) proteins. (2) During pulmonary infection, C. neoformans senses a high-Cu environment. Ctr1 is quickly degraded, but Ctr4 is still expressed. Cmt1 and Cmt2 are expressed to protect fungal cells from antimicrobial Cu in the host lung. (3) During meningoencephalitis, C. neoformans utilizes Ctr1 and Ctr4 for Cu uptake, whereas the expression of Cmt1 and Cmt2 is reduced and therefore these proteins play no function in the brain. We speculate that there are uncharacterized Cu transport machineries in C. neoformans , such as low-affinity or nonspecific transporters. ( b ) Models of the phenotypes of C. neoformans transporter mutants in vivo . (i) The wild-type strain degrades the Ctr1 Cu + transporter in the lung, while Ctr4 is active and transports the host antimicrobial Cu. (ii) In the brain, Ctr1 and Ctr4 are expressed for Cu acquisition. (iii and iv) In the ctr1Δ strain, the functionally redundant Cu+ transporter Ctr4 can transport Cu in both the lung and brain, enabling growth in both tissues similar to that observed for wild-type C. neoformans. (v) The ctr4Δ strain exhibits increased fungal proliferation in the lung due to the fast protein degradation of Ctr1 and the disruption of CTR4 , leading to increased dissemination of fungal cells into the brain. (vi) Because the functionally redundant Cu + transporter Ctr1 is expressed in ctr4Δ cells and the number of ctr4Δ cells in the brain is increased, the ctr4Δ strain exhibits increased fungal virulence. (vii) The cell growth of the ctr1Δctr4Δ strain is increased in the lung, resembling that of the ctr4Δ strain, resulting in increased dissemination of fungal cells in the brain. (viii) Owing to the lack of functional Cu + transporters in the ctr1Δctr4Δ strain, the cell growth is inhibited in the brain. Therefore, the Cu-replete environment in the lung and Cu-deficient conditions in the brain generates a Cu-balance for the ctr1Δctr4Δ strain, resulting in a survival rate equal to that of the wild type. Full size image Little is known about cryptococcal meningoencephalitis and brain immunity. In fact, the brain is a site of immune privilege, with unique immune responses compared with other tissues [46] . Brain immune cells must maintain a balance between killing invading microbes and preventing robust inflammatory responses to protect fragile neurons [46] . Despite the importance of microglial cells in protection against C. neoformans , the expression of brain proinflammatory cytokines (TNF-α, Interleukin (IL)-12 and IL-1) is low at the early stages of infection [47] . Furthermore, damage to the central nervous system causes inhibition of NF-κB in astrocytes, which, in turn, blocks the expression of a range of cytokines, including mammalian Cu transporter inducers, such as IFN-γ [48] . Our data demonstrated that the production of cytokines, including IFN-γ and TNF-α, is induced by C. neoformans infection in the lung tissues but not in the brain. Most importantly, Cu accumulation is often associated with neurodegenerative disease [49] . In conclusion, our study highlights the reciprocal roles of C. neoformans Cu transporters in the host, and underscores the importance of analysing host niches during the investigation of Cryptococcus pathogenicity. Strains and media The C. neoformans H99 strain was generously provided by Ying-Lien Chen (National Taiwan University). The ctr4Δ::URA5 strain was a gift from Dr Peter Williamson (National Institute Health, USA) to Dr Jia-Yi Li (Lund University, Sweden). All mutants ( Supplementary Table ) were routinely grown in YPD (1% yeast extract, 1% peptone and 2% dextrose) or synthetic complete (SC: 0.67% yeast nitrogen base, 2% dextrose and 0.2% amino acids) as previously described and generated as described below [5] . SC (114400022) and SC- ura dropout mixes (114410622) were purchased from MP Biomedicals. For biolistic transformation, YPD 2% agar supplemented with 1 mM sorbitol was used. For selection of transformants, nourseothricin or G418 was added to YPD at a final concentration of 100 μg ml −1 , and hygromycin B was added to YPD at a final concentration of 200 units ml −1 . Generation of Cryptococcus mutants CTR1 and CTR4 overexpression strains were generated as described below. The genomic DNA from CTR1 and CTR4 were amplified using primers (5′-GGGAACAAAAGCTGGAGCTCCCTTTGCGGAAGTAAAGAAGC-3′ and 5′-ATCCACTAGTTCTAGATCGAATGGCCAGTAAGGAACT-3′ for CTR1 , and 5′-GGGAACAAAAGCTGGAGCTCTTTGGTCGACAGAACAATCGG-3′ and 5′-ATCCACTAGTTCTAGAACATCCCTCGTCTCATCCAC-3′ for CTR4 . PCR products were cloned into the pHYG-7KB plasmid [50] , between the SacI and XbaI sites using the In-Fusion PCR cloning kit (Clontech). The cloned plasmids were used to transform C. neoformans strains by biolistic transformation [51] . Strains were isolated, and the RNA expression levels of CTR1 and CTR4 were confirmed using real-time PCR. The ura5Δ strain was generated by homologous recombination method. Primers 5′-NNNNCTCGAGTAGTCCTCAGTTTTTGATTCTACTTG-3′ and 5′-NNNNCCCGGGGATCAAGTTCTTATTTGGTCGCCGTTG-3′ were used to amplify the upstream sequence, and primers 5′-NNNNGGATCCAGGGTTTTCTTGGATGCAGGGGT-3′ and NNNNGAGCTCTCTCTCTCTCCCAAACCAAAGTCTC-3′ were used to amplify the downstream sequence. The PCR products were cloned into the pHYG plasmid (containing a hygromycin resistance marker under the control of the Cryptococcus ACT1 promoter), the upstream sequence was inserted between the XhoI and XmaI sites and the downstream sequence was inserted between the BamHI and SacI sites. The cloned plasmid was amplified using the primers 5′-NNNNCTCGAGTAGTCCTCAGTTTTTGATTCTACTTG-3′ and 5′-NNNNGAGCTCTCTCTCTCTCCCAAACCAAAGTCTC-3′ to generate a knockout cassette. The PCR product was then used to transform the wild-type H99 strain. Transformants were first tested for growth in the absence of uracil, and the integration of the knockout cassette was confirmed with Southern blott analysis. The ctr4Δ::URA5 strain was generated exactly as described previously [18] . The cmt1Δcmt2Δctr4Δ strain was generated as described previously [12] , except the hygromycin resistance marker was used. The HA integration cassette (pHA-NEO) was generated as described below. The primers 5′-NNNNCCCGGGTACCCATACGATGTTCCAGATTACGCTTAAGGGTTACAGTAGCAGTAGTAATG-3′ and 5′-CTCCAGCTCACATCCTCGCAGCTCTTCACGTGGACGCTCCAAGG-3′ were used to amplify the terminator sequence from GPD1 , and the primers 5′-GCTGCGAGGATGTGAGCTGGAG-3′ and 5′-NNNNGGATCCTTTAGGCCTAAGAGATGTAGAAACTAGCTTC-3′ were used to amplify the neomycin resistance marker. The two PCR products were then joined by overlapping PCR, and the resulting product was cloned into the pBluescript plasmid between the XmaI and BamHI sites. For genomic integration of an HA tag at the 3′ end of the gene of interests, the stop codons of CTR1 , CTR4 and CMT1 were deleted and replaced with the HA tag-TAA-GPD terminator-HYG marker construct ( Fig. 5a ). Briefly, downstream sequences (1 kb after the stop codon) were amplified using the primers 5′-NNGGATCCGGGGTGCGTATGTATGCATGT-3′ and 5′-NNTCTAGATCGAATGGCCAGTAAGGAACT-3′ for CTR1 , 5′-NNGGATCCAAGAGTAATAATATGTACCGGATGTTGATAG-3′ and 5′-NNTCTAGAAACATTACCTAGGATTCCCTATCCTCT-3′ for CTR4 , and 5′-NNGGATCCGCTTGTCTTCCAGACCAATG-3′ and 5′-NNGAGCTCCTTTTGAGAATGCCGAGAGG-3′ for CMT1 . The PCR products were then cloned into the pHA-NEO plasmid between the BamHI and XbaI sites for CTR1 and CTR4 , and the BamHI and SacI sites for CMT1 . Upstream sequences of CTR1 , CTR4 and CMT1 were amplified using the primers 5′-NNGGGCCCTGTCCTCTACATCCTCCAACA-3′ and 5′-ATGCCCAACATGACTTGACCC-3′ for CTR1 , 5′-NNGGGCCCGACATGGGTAACATGGGCAT-3′ and 5′-ACAACAGCGCCCCTGAGCAC-3′ for CTR4 , and 5′-NNCTCGAGAGAACACATCTGCATCCGATA-3′ and 5′-GGCAGCGCCAGATCCGCTGC-3′ for CMT1 . The PCR products were then cloned into the pHA-NEO plasmid, between the ApaI and SmaI sites for CTR1 and CTR4 , and the XhoI and SmaI sites for CMT1 . The integration cassettes were then amplified, and the resulting PCR products were used to transform the wild-type H99 strain. Transformants were tested by diagnostic PCR, and correct integrations of the HA tag were confirmed with western blot analysis. The CTR4 open reading frame was mutated by PCR ( Supplementary Fig. 6A ). CTR4 genomic DNA was amplified using two primer pairs 5′-NNNNCTCGAG TTGTTTTGGTCCGTTGA -3′ and 5′-CATGTGGCTGTGCTGGTGGCCGGAGTCCATACCCATGCCCATGCC-3′, and 5′-CCGGCCACCAGCACAGCCACATG-3′ and 5′-NNNNCCCGGGTTAAGCGTAATCTGGAACATCGTATGGGTAACAACAGCGCCCCTGAGCAC-3′. The resulting two PCR products were joined by overlapping PCR, and the resulting product was clond into the CTR4HA integration cassette, to replace the CTR4 upstream sequence. The cloned plasmid was sequenced to confirm the mutated codon. The correct mutation plasmids were then amplified to generate integration cassettes, which were used to transform ctr1Δctr4Δ cells. Correct integrations were confirmed by diagnostic PCR, followed by spotting assays and western blots. Capsule formation and release Cells were grown overnight in SC medium and then washed three times with H 2 O. The cells were resuspended in RPMI medium supplemented with 10% fetal calf serum (FCS) and incubated for 3 days at 37 °C, 5% CO 2 . Capsule release experiments were performed as previously described [52] . Briefly, capsule release was induced in RPMI medium supplemented with 10% FCS for 5 days at 37 °C, 5% CO 2 . One millilitre aliquot of cell culture was removed and incubated at 70 °C to denature enzymes. The resulting supernatant samples were filtered using a 0.2-μm filter to remove fungal cells, followed by separation in an agarose gel at 4 °C and 25 V overnight. The capsule molecules were then transferred on a nylon membrane. Immunoblotting was performed using the monoclonal antibody 18B7 at a 1:1,000 dilution [53] . Biofilm formation Cryptococcus cells were grown in SC medium overnight at 30 °C. The cells were then washed three times with PBS and resuspended to an A 600 of 1.0 in SC medium. The cell culture (100 μl) was transferred to 96-well plates, and the plates were incubated at 37 °C for 24 h. Each well was washed with PBS five times to remove non-adherent cells. A 100-μl aliquot of 0.1% crystal violet solution was added into each well and incubated for 15 min at 30 °C. Excess crystal violet was washed five times with PBS. A 100-μl aliquot of 30% glacial acetic acid was added and incubated for 4 h to release the crystal violet dye from the biofilm structure. Biofilm production was then quantified by measuring the absorbance of the released crystal violet dye at 570 nm. Nucleic acid isolation and real-time PCR DNA was isolated as previously described [38] . Briefly, 5 ml of an overnight Cryptococcus cell culture in YPD was washed with water and resuspended in lysis buffer (10 mM Tris-HCl, pH 8.0, 1 mM EDTA, 100 mM NaCl, 1% SDS, 2% Triton-X). Cells were lysed using a bead beater. The supernatant was mixed with 275 μl of 7 M ammonium acetate for 5 min at 65 °C. The DNA was precipitated with isopropanol, washed with 70% ethanol and resuspended in 50 μl of H 2 O supplemented with RNase A. One microgram of genomic DNA was used for PCR, and 20 μg of genomic DNA was used for Southern blot analysis. RNA was isolated using the TRIzol reagent (Life Technologies), and Turbo DNase I (Life Technologies) was used to eliminate genomic DNA contamination. One microgram of total RNA was used for cDNA synthesis, using the GoScript Reverse Transcription System (A5001, Promega), and real-time PCR was performed using a CFX Connect Thermocycler (Bio-rad) as previously described [5] . RNA was isolated from mice infected with C. neoformans as previously described [30] . Briefly, infected lung tissues were first cut into small pieces and resuspended in TRIzol reagent. Glass beads were added, and the mixture was processed using a bead beater. The gene copy number of Ctr4 glycosylation mutants was characterized using real-time PCR as previously described [54] . Animal and human CSF CFU experiments All animal experiments were reviewed and ethically approved by the Research Ethics Committees of the College of Life and Health Sciences of Northeastern University. Six- to eight-week-old female A/J and C57BL/6 mice were purchased from the National Cancer Institute (USA) and Changsheng Biotech (China), respectively, and used for infection and fungal burden assays. Intranasal and intracerebral infections were performed as previously described [5] , [55] . For intranasal infections, mice were anaesthetized and intranasally infected with 10 5 fungal cells in 50 μl PBS. For intracerebral infections, mice were anaesthetized and Cryptococcus cells in 3 μl of PBS were injected into lateral ventricle using a mouse brain stereotactic instrument. Fungal burden assays were performed as described below. Infected mice were killed by exposure to CO 2 for 5 min. Lung and brain tissues were isolated, weighed and placed in 5 ml of PBS buffer. The tissues were then homogenized, and the suspension was plated on SC agar at 30 °C for 3 days. For immunohistochemistry, tissues were isolated and fixed in paraformaldehyde. Fixed tissues were frozen and tissues sections (10-μm thick) were processed using a Crypstat Microtome Leica CM1850 (Leica). Immunohistochemistry and haematoxylin and eosine staining were performed as previously described [5] . TUNEL staining was performed according to the manufacturer’s instructions (Roche). The human CSF sample was kindly provided by Dr Hao Zhang, MD (China Medical University). The CSF samples were pooled from three patients, each with a written formal consent. The utilization of human CSF samples was reviewed and ethically approved by the Laboratory Ethics Committees of China Medical University and the Research Ethics Committees of the College of Life and Health Sciences of Northeastern University. The CFU in human CSF was performed as described previously [56] . Protein quantifications and SOD activity measurements Immunoblotting signals were captured using ChemiDoc XRS+ (Bio-Rad). Anti-HA (ab9110, Abcam; 1:1,000 dilution) and anti-histone H3 antibodies (4499P, Cell Signaling; 1:1,000 dilution) were used. The Protein Deglycosylation Mix kit (P6039S, NEB) was used as described in the manufacturer’s manual. Briefly, an overnight culture of fungal cells were subcultured in SC medium supplemented with 1 mM BCS for 6 h at 30 °C. The cells were resuspended in HEPES buffer (50 mM HEPES, 140 mM NaOH, 1% Tritone X-100, 1 mM EDTA and protease inhibitors). Proteins were isolated using a bead beater and incubated with the deglycosylation enzyme mixture for 4 h at 37 °C under denaturing conditions or nondenaturung condition according to the manual of Protein Deglycosylation Enzyme kit (NEB). The reaction mixtures were then separated by 15% SDS–PAGE. Immunoblottings were then performed using the HA antibody. Mouse IFN-γ (ELM-IFNg) and TNF-α (ELM-TNFa) ELISA kits were purchased from RayBiotech, and experiments were performed according to the manufacturer’s instructions. The SOD activity was quantified using the SOD activity kit (Jiancheng Bio) according to the manufacturer’s instructions. Cryptococcus indirect immunofluorescent microscopy The immunofluorescent microscopy was performed as described previously [12] . Cells were grown in SC medium overnight and then subcultured for additional 3 h in the presence of 100 μM BCS to induce protein expression levels of Ctr4HA and N19Q mutant. Formaldehyde was then added to fix the cells, and the cells were incubated at 4 °C for 1 h with gentle shaking. The cells were then washed with PBS and resuspended in sorbitol buffer. Lysing enzyme (L1214, Sigma) supplemented with protease inhibitor (Roche) was used to digest the cell wall at 37 °C. Cells were then washed with PBS and resuspended in a PBS BSA solution and adhered to a glass slide treated with poly-lysine. The anti-HA antibody (1:300) was added and incubated at 4 °C overnight, followed by washing with the PBS BSA solution. Secondary antibody (conjugated Alexa flour 488) was added and incubated at room temperature for 30 min. The slides were washed, mounted and observed using a LEICA DM6000CS microscope. Microscopy analysis Two-photon microscopy was performed using an LSM 7MP (Zeiss). After infection, tissues were removed and examined to identify GFP fluorescent signals. All images were acquired with the × 10 lens, and brain images were further magnified four times using the CROP function of the ZEN2012 software (Zeiss). All images were quantified using ZEN2012. How to cite this article : Sun, T.-S. et al. Reciprocal functions of Cryptococcus neoformans copper homeostasis machinery during pulmonary infection and meningoencephalitis. Nat. Commun. 5:5550 doi: 10.1038/ncomms6550 (2014).